Organellar mechanosensitive channels in fission yeast regulate the hypo-osmotic shock response A key molecule of sensing machineries essential for survival upon hypo-osmotic shock is the mechanosensitive channel. The bacterial mechanosensitive channel MscS functions directly for this purpose by releasing cytoplasmic solutes out of the cell, whereas plant MscS homologues are found to function in chloroplast organization. Here we show that the fission yeast MscS homologues, designated Msy1 and Msy2, participate in the hypo-osmotic shock response by a mechanism different from that operated by the bacterial MscS. Upon hypo-osmotic shock, msy2 – and msy1 – msy2 – cells display greater cell swelling than wild-type cells and undergo cell death. Cell swelling precedes an intracellular Ca 2+ increase, which was greater in msy1 – and msy1 – msy2 – cells than in wild-type cells. Fluorescent microscopy showed that Msy1 and Msy2 localize mainly to the endoplasmic reticulum. These observations suggest that organellar Msy1 and Msy2 regulate intracellular Ca 2+ and cell volume for survival upon hypo-osmotic shock. Living cells regulate their own cell volume when challenged by osmotic environmental changes. Upon hypo-osmotic shock, cell swelling is followed by volume regulation to prevent the collapse of ion homoeostasis and cell injury by the sudden increase in cell volume. The mechanisms of the hypo-osmotic shock response have been studied mainly in mammalian and bacterial cells. The mammalian cells are triggered by Ca 2+ influx through mechanosensitive transient receptor potential channels upon cell swelling [1] , [2] , [3] . A transient increase in intracellular Ca 2+ concentration opens Ca 2+ -activated K + and Cl − channels to reduce osmotic gradients and activates a stress-response MAP kinase cascade [4] . By contrast, the hypo-osmotic shock response in bacterial cells is conducted exclusively by mechanosensitive channels and does not require such a secondary messenger system. In Escherichia coli , three discrete types of mechanosensitive channels, MscM, MscS and MscL, are activated by cell swelling, and release ions and small osmolytes non-selectively to reduce the intracellular osmolarity [5] , [6] . Genes encoding MscS homologues have been found in the genomes of prokaryotes and cell-walled eukaryotes, (for example, plants, algae and fungi) [7] . While MscS is required for the osmotic response in bacteria [6] , [8] , [9] , it is unknown whether eukaryotic MscS homologues are involved in the osmotic response. Rather, eukaryotic MscS homologues analyzed so far, such as Arabidopsis thaliana MscS-like proteins MSL2 and MSL3 and Chlamydomonas reinhardtii MscS homologue MSC1, are associated with chloroplast organization [10] , [11] . Interestingly, MSL2, MSL3 and MSC1 are expressed in organellar membranes, including the chloroplast. However, chloroplast organization cannot be the only function of MscS homologues because they are also present in fungal genomes. Yeast cells may have osmotic response mechanisms similar to mammalian cells because they generate a Ca 2+ increase upon hypo-osmotic shock [12] . It is unclear, however, whether the Ca 2+ increase is correlated to cell volume regulation and what channels are responsible for the Ca 2+ increase. In this study, we report that two MscS homologues in fission yeast (Msy1 and Msy2) are organellar mechanosensitive channels required for the hypo-osmotic shock response. We found that msy2 – and msy1 – msy2 – mutants exhibit an excessive increase in cell volume upon hypo-osmotic shock. The cell swelling was accompanied by an increase in intracellular Ca 2+ concentration and this increase was abnormally high in the msy1 – and msy1 – msy2 – mutants. These results suggest that Msy1 and Msy2 regulate intracellular Ca 2+ levels and cell volume upon hypo-osmotic shock in fission yeast. Evolutionary relationship of MscS homologues in fungi Two MscS homologues were found in the S. pombe genome by a BLAST search against E. coli MscS and were designated Msy1 and Msy2. The amino-acid sequences of Msy1 and Msy2 display a total of 52.7% similarity ( Supplementary Fig. S1 ). Homologues of Msy1 were found in the genomes of a wide range of ascomycetes and basidiomycetes, but not in the Saccharomyces cerevisiae genome, which contains a mechanosensitive transient receptor potential channel [13] TrpY1, and another as-yet-unidentified mechanosensitive channel [14] . We performed a phylogenetic analysis based on maximum likelihood with sequences corresponding to the MscS domain (Accession code COG0668) defined in the conserved domain database of the National Center for Biotechnology Information. Although MscS homologues of plants, algae and bacteria did not diverge into discrete branches, MscS homologues of fungi fell into a single discrete cluster ( Fig. 1a ), suggesting that the MscS homologues of fungi are conserved more closely than those of plants, algae and bacteria. 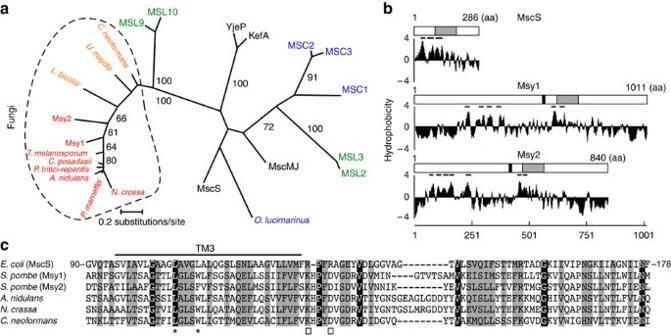Figure 1: Evolutionary feature of fungal MscS homologues. (a) Phylogenetic tree for MscS family created with the maximum likelihood method. Dashed line shows the fungal MscS homologues. Colours represent prokaryotes (black), ascomycetes (red), basidiomycetes (orange), algae (blue) and land plants (green). Bootstrap proportions (BPs) with 100 repetitions are shown. Unmarked branches have <60 BP. The UniProt accession numbers are P11666 (E. coli, MscS), P77338 (E. coli, KefA), P39285 (E. coli, YjeP), Q57634 (M. jannaschii, MscMJ), ABP00956 (O.lucimarinus), BAF48401 (C. reinhardtii, MSC1), XP_001690099 (C. reinhardtii, MSC2), XP_001689635 (C. reinhardtii, MSC3), NP_568230 (A. thaliana, MSL2), NP_974046 (A. thaliana, MSL3), NP_197453 (A. thaliana, MSL9), NP_196769 (A. thaliana, MSL10), NP_587894 (S. pombe, Msy1), NP_594520 (S. pombe, Msy2), XP_680840 (A. nidulans), EER23643 (C. posadasii), XP_961167 (N. crassa), XP_002149714 (P. marneffei), XP_001938146 (P. tritici-repentis), XP_002840873 (T. melanosporum), XP_776457 (C. neoformans), XP_001877365 (L. bicolor), XP_758384 (U. maydis). (b) Structural features of Msy1 and Msy2. The hydrophobicity plot was generated according to Kyte and Doolittle45. Bars indicate the transmembrane segments predicted by the TMHMM program46. Black and grey boxes show an EF hand-like motif and an MscS family-conserved domain, respectively. (c) Alignment of domains conserved betweenE. coliMscS and fungal MscS homologues. Fungal MscS homologues were aligned in the sequence corresponding to the third transmembrane region and the adjacent conserved sequence ofE. coliMscS. Identical residues are highlighted in black and similar residues are shown in grey. L105 and L109 that form a pore constriction in MscS are indicated with asterisks. R128 and R131 involved in salt bridges are shown with squares. Figure 1: Evolutionary feature of fungal MscS homologues. ( a ) Phylogenetic tree for MscS family created with the maximum likelihood method. Dashed line shows the fungal MscS homologues. Colours represent prokaryotes (black), ascomycetes (red), basidiomycetes (orange), algae (blue) and land plants (green). Bootstrap proportions (BPs) with 100 repetitions are shown. Unmarked branches have <60 BP. The UniProt accession numbers are P11666 ( E. coli , MscS), P77338 ( E. coli , KefA), P39285 ( E. coli , YjeP), Q57634 ( M. jannaschii , MscMJ), ABP00956 (O. lucimarinus ), BAF48401 ( C. reinhardtii , MSC1), XP_001690099 ( C. reinhardtii , MSC2), XP_001689635 ( C. reinhardtii , MSC3), NP_568230 ( A. thaliana , MSL2), NP_974046 ( A. thaliana , MSL3), NP_197453 ( A. thaliana , MSL9), NP_196769 ( A. thaliana , MSL10), NP_587894 ( S. pombe , Msy1), NP_594520 ( S. pombe , Msy2), XP_680840 ( A. nidulans ), EER23643 ( C. posadasii ), XP_961167 ( N. crassa ), XP_002149714 ( P. marneffei ), XP_001938146 ( P. tritici-repentis ), XP_002840873 ( T. melanosporum ), XP_776457 ( C. neoformans ), XP_001877365 ( L. bicolor ), XP_758384 ( U. maydis ). ( b ) Structural features of Msy1 and Msy2. The hydrophobicity plot was generated according to Kyte and Doolittle [45] . Bars indicate the transmembrane segments predicted by the TMHMM program [46] . Black and grey boxes show an EF hand-like motif and an MscS family-conserved domain, respectively. ( c ) Alignment of domains conserved between E. coli MscS and fungal MscS homologues. Fungal MscS homologues were aligned in the sequence corresponding to the third transmembrane region and the adjacent conserved sequence of E. coli MscS. Identical residues are highlighted in black and similar residues are shown in grey. L105 and L109 that form a pore constriction in MscS are indicated with asterisks. R128 and R131 involved in salt bridges are shown with squares. Full size image Msy1 and Msy2 are composed of an extended N-terminal segment, six predicted transmembrane segments and a putative C-terminal cytoplasmic domain. In contrast to MscS homologues of Arabidopsis and Chlamydomonas , Msy1 and Msy2 do not have predicted signal sequences in the extended N-terminal segment but have an EF hand-like motif in the middle of the entire sequences ( Fig. 1b ). The EF hand-like motif was found to be present exclusively in all fungal MscS homologues surveyed ( Table 1 ). Table 1 Conservation of EF hand-like motif in fungal MscS homologs. Full size table Fungal MscS homologues have the highest degree of homology in the region that corresponds to the pore-forming transmembrane segment (TM3) and the upper roof of the cytoplasmic vestibule [15] . In this region, the amino-acid sequences of Msy1 and Msy2 have 25.8% and 21.3% identity, respectively, to that of E. coli MscS. Residues in this region, which are structurally and functionally important in E. coli MscS, are not well conserved in fungal MscS homologues. Firstly, G104 and G108 of E. coli MscS, needed for close packing of TM3 helices [16] , and G113 and G121, necessary for the kinks of the TM3 helices [17] , are replaced with amino acids with side chains ( Fig. 1c ). These changes may alter inactivation kinetics as observed in G113A and G121A mutants [17] . Secondly, whereas L105, one of the leucine residues that form hydrophobic seals at the pore of E. coli MscS, is totally conserved among fungal MscS homologues, another leucine residue, L109, is substituted with aromatic amino acids. The change at L109 possibly alters mechanosensitivity, as was observed in L109S MscS [18] . Lastly, R131, one of two arginine residues that coordinate the movement of the transmembrane segment with that of the cytoplasmic vestibule through formation of a salt bridge [19] , is substituted with a residue with opposite charge in fungi although the other arginine residue, R128, is replaced with an amino acid with the same charge, Lys. Like R131D mutant [19] , the changes in the charge at these positions would affect both mechanosensitivity and the inactivation rate. Subcellular localization of Msy1 and Msy2 Because the MscS homologues analyzed physiologically so far are localized to the chloroplast [10] , [11] , [20] , we determined the localization of Msy1. The chromosomal msy1 + gene was replaced with a four-hemagglutinin (HA)-tagged msy1 + by homologous recombination. Western blotting showed that the anti-HA antibody recognized a specific, predicted Msy1-4HA band of 140 kDa ( Fig. 2a ). Indirect immunofluorescence microscopy with an anti-HA antibody revealed that the majority of fluorescent signals from Msy1-4HA were present as punctate spots in the periphery of the DAPI-stained nucleus ( Fig. 2b ). The signals of Msy1 overlapped with those of binding immunoglobulin protein (BiP), which is localized to the perinuclear endoplasmic reticulum (ER) [21] . No signal was observed when the primary antibody was omitted. The localization of the periphery of the nucleus was consistent with a report in the S. pombe Postgenome Database ORFeome Localization Data (29/29H05) [22] . Because we failed to detect Msy2 by the same procedure, we fused mCherry at the N-terminus of Msy2. The signals of the mCherry-Msy2 fusion protein overlapped with those of calnexin (Cnx)-EGFP, an ER marker [23] ( Fig. 2c ), suggesting that Msy2 is localized in the cortical ER. To confirm this suggestion, we examined whether the signal of mCherry-Msy2 overlaps with that of reticulon-like protein (Rtn1)-EGFP, a cortical ER marker [24] and plasma-membrane proton-efflux P-type ATPase (Pma1)-EGFP, a plasma membrane marker [25] . The signals of mCherry-Msy2 generally merged with the signals of Rtn1-EGFP. On the other hand, signals of Pma1-EGFP did not merge and localized to the periphery of the signals of mCherry-Msy2 ( Fig. 2d ), suggesting that Msy2 is localized in the cortical ER rather than the plasma membrane. We confirmed that Msy1 and Msy2 tagged with HA and mCherry rescued msy1 – msy2 – cells from hypo-osmotic shock-induced cell death, suggestive of their functional localization ( Fig. 2e ). 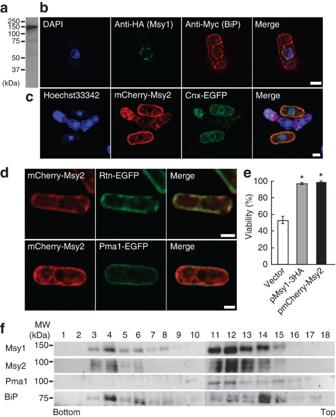Figure 2: Subcellular localizations of Msy1 and Msy2. (a) Western blots of whole-cell extracts for Msy1-4HA. (b) Immunofluorescence images of DAPI (blue), Msy1-4HA (green) and BiP-myc (red). Yellow signals in the merged image show the overlap of Msy1-4HA and Bip-myc. (c) Fluorescence confocal images of Hoechst33342 (blue), Calnexin-EGFP (green) and mCherry-Msy2 (red). Yellow signals in the merged image show the overlap of mCherry-Msy2 and Calnexin-EGFP. (d) Fluorescence confocal images of Rtn1-EGFP (green), Pma1-EGFP (green) and mCherry-Msy2 (red). Yellow signals in the merged image show the overlap of mCherry-Msy2 and Rtn1-EGFP. Scale bars indicate 2 μm. (e) Complementation of the phenotype ofmsy1–msy2–cells by the expression of taggedmsy1+andmsy2+under the control of thenmt41promoter on pREP41. Cells were precultured overnight in EMM2 medium containing 1.2 M sorbitol, diluted 20-fold with distiled water to apply hypo-osmotic shock, and incubated further for 30 min. The viability was examined with methylene blue and the ratio of the number of viable cells to the total number of cells including non-viable cells was used to represent viability: empty vector (white),msy1+-3HA(grey),mCherry-msy2+(black). Error bars represent the s.d. of three independent experiments. *, Student'st-test,P<0.05 versus the empty vector. (f) Subcellular fractionation using sucrose density gradient centrifugation. Pma1 and BiP were used as the plasma membrane and ER markers, respectively. Strain FY15952 was used as a host for all the plasmids carrying the tagged proteins described above. Figure 2: Subcellular localizations of Msy1 and Msy2. ( a ) Western blots of whole-cell extracts for Msy1-4HA. ( b ) Immunofluorescence images of DAPI (blue), Msy1-4HA (green) and BiP-myc (red). Yellow signals in the merged image show the overlap of Msy1-4HA and Bip-myc. ( c ) Fluorescence confocal images of Hoechst33342 (blue), Calnexin-EGFP (green) and mCherry-Msy2 (red). Yellow signals in the merged image show the overlap of mCherry-Msy2 and Calnexin-EGFP. ( d ) Fluorescence confocal images of Rtn1-EGFP (green), Pma1-EGFP (green) and mCherry-Msy2 (red). Yellow signals in the merged image show the overlap of mCherry-Msy2 and Rtn1-EGFP. Scale bars indicate 2 μm. ( e ) Complementation of the phenotype of msy1 – msy2 – cells by the expression of tagged msy1 + and msy2 + under the control of the nmt41 promoter on pREP41. Cells were precultured overnight in EMM2 medium containing 1.2 M sorbitol, diluted 20-fold with distiled water to apply hypo-osmotic shock, and incubated further for 30 min. The viability was examined with methylene blue and the ratio of the number of viable cells to the total number of cells including non-viable cells was used to represent viability: empty vector (white), msy1 + - 3HA (grey), mCherry - msy2 + (black). Error bars represent the s.d. of three independent experiments. *, Student's t -test, P <0.05 versus the empty vector. ( f ) Subcellular fractionation using sucrose density gradient centrifugation. Pma1 and BiP were used as the plasma membrane and ER markers, respectively. Strain FY15952 was used as a host for all the plasmids carrying the tagged proteins described above. Full size image We also performed membrane fractionation by sucrose density gradient centrifugation to confirm the localization of Msy2. The distribution pattern of Msy2 was similar to that of BiP on the gradients ( Fig. 2f ). Taken together, these observations suggest that Msy1 and Msy2 are mainly targeted to the perinuclear and cortical ERs, respectively. Msy1 and Msy2 are required for hypo-osmotic shock survival We generated chromosomal gene deletion mutants of msy1 + and msy2 + , and their disruption was verified by PCR with reverse transcription (RT–PCR) ( Fig. 3a ). To examine the involvement of Msy1 and Msy2 in the osmotic response, cells of the wild type (WT), msy1 – , msy2 – and msy1 – msy2 – were subjected to hypo-osmotic shock. A wide range of hypo-osmotic shock was applied by preincubating the cells in YES medium supplemented with 0–1.5 M sorbitol, and then diluting the culture medium into distiled water and incubating for a further 30 min. WT cells tolerated this hypo-osmotic shock and showed viability as high as 90% over the entire sorbitol concentration range ( Fig. 3b ). By contrast, the viability of the msy1 – msy2 – mutant was reduced with increases in the magnitude of hypo-osmotic shock and reached ~50% with downshocks from YES medium supplemented with 1.2 and 1.5 M sorbitol ( Fig. 3b ). The decrease in viability was also observed in msy2 – , although the degree was smaller. The viability of msy1 – cells was not significantly different from that of WT cells. The decreased viability was not owing to cell death during preincubation in sorbitol because viability did not decrease in the absence of osmotic downshock. This observation suggests that Msy1 and Msy2 are required for survival upon hypo-osmotic shock. Plasmid-based expression of msy1 + or msy2 + restored the viability of the msy1 – msy2 – mutant to the WT level ( Fig. 3c ), indicating that the phenotype of the msy1 – msy2 – mutant is caused by the disruption of Msy1 and Msy2. 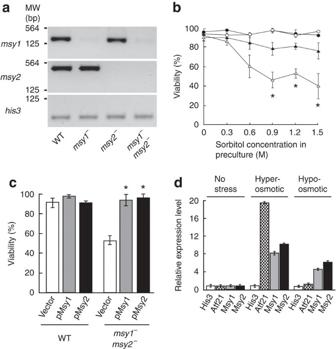Figure 3: Physiological functions of Msy1 and Msy2. (a) Confirmation of gene disruptant using RT–PCR. (b) Relationship between viability and the amplitude of hypo-osmotic shock. Symbols show the wild type (closed circle),msy1–mutant (open circle),msy2–mutant (closed triangle) andmsy1–msy2–mutant (open triangle). Cells were precultured overnight in YES medium containing 0, 0.3, 0.6, 0.9, 1.2 and 1.5 M sorbitol, diluted 20-fold with distiled water to give hypo-osmotic shock, and incubated further for 30 min. *, Student'st-test,P<0.05 versus wild type. (c) Rescue of the phenotype ofmsy1–msy2–mutant by the expression ofmsy1+andmsy2+under thenmt41promoter on pREP41. The viability of cells was examined as described in the legend toFig. 2e: empty vector (white),msy1+(grey),msy2+(black). *, Student'st-test,P<0.05 versus empty vector. (d) Quantitative real-time PCR on RNA that was extracted from cells subjected to either hyper- or hypo-osmotic shock for 30 min.Atf21was used as a positive control for hyper-osmotic shock.His3was used as a negative control. The expression levels are normalized by those without shock. All of the data are means±s.d. from three independent experiments. Figure 3: Physiological functions of Msy1 and Msy2. ( a ) Confirmation of gene disruptant using RT–PCR. ( b ) Relationship between viability and the amplitude of hypo-osmotic shock. Symbols show the wild type (closed circle), msy1 – mutant (open circle), msy2 – mutant (closed triangle) and msy1 – msy2 – mutant (open triangle). Cells were precultured overnight in YES medium containing 0, 0.3, 0.6, 0.9, 1.2 and 1.5 M sorbitol, diluted 20-fold with distiled water to give hypo-osmotic shock, and incubated further for 30 min. *, Student's t -test, P <0.05 versus wild type. ( c ) Rescue of the phenotype of msy1 – msy2 – mutant by the expression of msy1 + and msy2 + under the nmt41 promoter on pREP41. The viability of cells was examined as described in the legend to Fig. 2e : empty vector (white), msy1 + (grey), msy2 + (black). *, Student's t -test, P <0.05 versus empty vector. ( d ) Quantitative real-time PCR on RNA that was extracted from cells subjected to either hyper- or hypo-osmotic shock for 30 min. Atf21 was used as a positive control for hyper-osmotic shock. His3 was used as a negative control. The expression levels are normalized by those without shock. All of the data are means±s.d. from three independent experiments. Full size image To examine the possibility that msy1 + and msy2 + are transcriptionally induced by hyper- and hypo-osmotic shock like E. coli MscS [26] , we assessed the levels of msy1 + and msy2 + transcripts using quantitative real-time PCR after cells were transferred from YES medium to YES medium supplemented with 1.2 M sorbitol, or distiled water. Because YES medium contains 167 mM D -glucose, transfer from YES medium to distiled water involves a hypo-osmotic shock greater than 167 mOsm. At 30 min after the transfer to YES medium with 1.2 M sorbitol, the levels of msy1 + and msy2 + transcripts increased approximately 8- to 10-fold relative to those in YES medium ( Fig. 3d ). A positive control, ATF/CREB-family transcription factor Atf21 (ref. 27 ), also showed an increase in expression. Similarly, 30 min after the transfer to distiled water, the levels of the msy1 + and msy2 + transcripts increased approximately fivefold. Therefore, the expressions of msy1 + and msy2 + are upregulated upon both hyper- and hypo-osmotic shocks. msy1 – msy2 – undergoes osmotic stress-induced cell death Upon hypo-osmotic shock, mammalian cells undergo osmotic stress-induced death, such as necrosis [28] , whereas prokaryotic cells experience cell lysis [6] . Thus, to examine whether the decreased viability of msy2 – cells and msy1 – msy2 – cells is due to osmotic-induced cell death or cell lysis, we performed a time-lapse imaging analysis with cells that express EGFP to monitor cell lysis. WT and mutant cells expressing EGFP showed fluorescence in the cytosol and the nucleus, but not in the vacuole. When WT and msy1 – cells were subjected to hypo-osmotic shock, cell volume was increased up to approximately 110% of the original volume and reached a plateau ( Fig. 4a , Supplementary Movies 1 and 2 ). On the other hand, msy2 – and msy1 – msy2 – cells swelled more extensively than WT cells, but after this 'overshoot', the cell volume was reduced significantly ( Fig. 4a , Supplementary Movies 3 and 4 ). The nucleus of WT and mutant cells swelled in the same proportion as the whole-cell volume, suggestive of an increase of membrane tension in the intracellular space ( Fig. 4b ). Importantly, when exposed to hypo-osmotic shock, msy2 – and msy1 – msy2 – cells still retained EGFP fluorescence, while WT cells treated with Zymolyase, which digests cell walls, lost EGFP fluorescence readily following hypo-osmotic shock ( Supplementary Movie 5 ), indicating that the cell death of msy1 – msy2 – cells is not due to cell lysis. To elucidate when the decrease of viability in msy1 – msy2 – cells occurs, we examined the time course of viability following hypo-osmotic shock. The viability of msy1 – msy2 – cells decreased gradually for about 30 min after hypo-osmotic shock, whereas that of WT cells did not change for 60 min ( Fig. 4c ). This time course is significantly slower than that of bacterial cell swelling (50 ms) and lysis (150–200 ms) [29] . These observations indicate that msy1 – msy2 – cells are defective in cell volume regulation, and that the decreased viability is caused by osmotic stress-induced cell death rather than cell lysis. 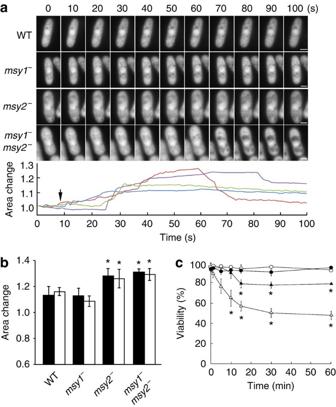Figure 4: Time-lapse observation of WT and mutant cells upon hypo-osmotic shock. (a) Cells expressing EGFP were incubated in EMM2 medium supplemented with 1.2 M sorbitol and diluted 20-fold with distiled water under microscopy. Photographs are displayed for every 10 s after the dilution. Scale bars indicate 2 μm (top). Relative cell volume changes of WT (blue),msy1–(green),msy2–(purple) andmsy1–msy2–(red) are shown (bottom). Arrow shows the application of hypo-osmotic shock with distiled water. (b) Maximum volume change of the entire cell (white) and the nucleus (black) in WT and mutant cells upon hypo-osmotic shock. (c) Time course of viability after hypo-osmotic shock. Symbols are the same as inFig. 3b. *, Student'st-test,P<0.05 versus wild type. All of the data are means±s.d. from three independent experiments. Figure 4: Time-lapse observation of WT and mutant cells upon hypo-osmotic shock. ( a ) Cells expressing EGFP were incubated in EMM2 medium supplemented with 1.2 M sorbitol and diluted 20-fold with distiled water under microscopy. Photographs are displayed for every 10 s after the dilution. Scale bars indicate 2 μm (top). Relative cell volume changes of WT (blue), msy1 – (green), msy2 – (purple) and msy1 – msy2 – (red) are shown (bottom). Arrow shows the application of hypo-osmotic shock with distiled water. ( b ) Maximum volume change of the entire cell (white) and the nucleus (black) in WT and mutant cells upon hypo-osmotic shock. ( c ) Time course of viability after hypo-osmotic shock. Symbols are the same as in Fig. 3b . *, Student's t -test, P <0.05 versus wild type. All of the data are means±s.d. from three independent experiments. Full size image Cell swelling induces an increase in intracellular Ca 2+ We monitored a change in intracellular Ca 2+ concentration ([Ca 2+ ] i ) with a Ca 2+ sensor yellow Cameleon-nano15 (ref. 30 ) to investigate the correlation between a [Ca 2+ ] i change and the cell volume increase upon hypo-osmotic shock. Upon hypo-osmotic shock with 10 mM CaCl 2 , a [Ca 2+ ] i elevation was observed approximately 20 s after the addition of the shock in both WT and mutant cells ( Fig. 5a , Supplementary Movies 6–9 ). Interestingly, this elevation was induced when cell volume increase reached a certain level before reaching its maximum level. The [Ca 2+ ] i elevation started in the entire cell or at the pole of cells, and spread over the intracellular space, including the nucleus. The [Ca 2+ ] i elevation in WT and msy1 – cells was sustained for 1–2 min, whereas [Ca 2+ ] i in msy2 – and msy1 – msy2 – cells decreased within 1 min. The degree of the [Ca 2+ ] i elevation in msy1 – and msy1 – msy2 – cells was greater than that in WT and msy2 – cells. Notably, the [Ca 2+ ] i elevation was quick and transient in msy1 – msy2 – cells, whereas it was relatively slow and durable in msy1 – cells, which did not show the overshoot of cell volume. Finally, we examined, using a Ca 2+ chelator, BAPTA (10 mM), whether extracellular Ca 2+ affects the overshoot in msy1 – msy2 – cells. Hypo-osmotic shock with this reagent did not affect the overshoot of cell volume ( Fig. 5b ), suggesting that the [Ca 2+ ] i increase is not the cause of the overshoot. These results indicate that the [Ca 2+ ] i increase is induced by cell swelling upon hypo-osmotic shock. 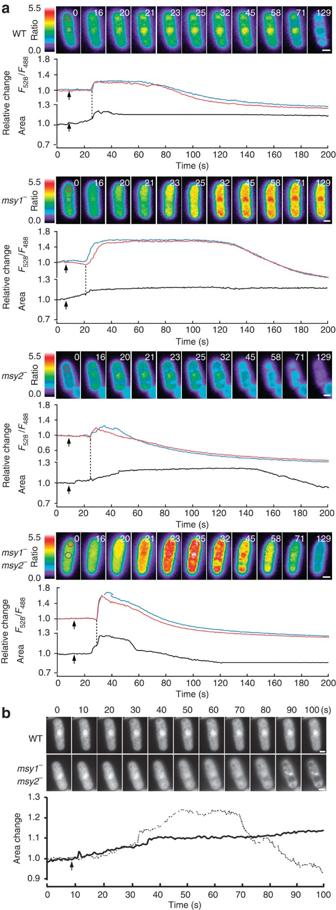Figure 5: Change of cell volume and intracellular Ca2+levels upon hypo-osmotic shock. (a) Ca2+imaging was performed with yellow Cameleon-nano15. Time-lapse photographs were taken at 0.5 s intervals in WT and mutant cells following hypo-osmotic shock with 10 mM CaCl2. Arrow indicates application of hypo-osmotic shock. White numbers show times (s) from application of hypo-osmotic shock. Solid lines show Ca2+change in the cytoplasm (red) and the nucleus (blue) and cell volume (black). Dashed lines show the start of increase in Ca2+level. Scale bars indicate 2 μm. (b) Time-lapse observation of WT andmsy1–msy2–cells upon hypo-osmotic shock with BAPTA. Cells expressing EGFP were incubated in EMM2 medium supplemented with 1.2 M sorbitol and diluted 20-fold with 10 mM BAPTA. Photographs are displayed for every 10 s after the dilution (top). Relative cell volume changes in WT andmsy1–msy2–cells are shown by solid and dashed lines, respectively (bottom). An arrow shows the application of hypo-osmotic shock. Scale bars indicate 2 μm. Figure 5: Change of cell volume and intracellular Ca 2+ levels upon hypo-osmotic shock. ( a ) Ca 2+ imaging was performed with yellow Cameleon-nano15. Time-lapse photographs were taken at 0.5 s intervals in WT and mutant cells following hypo-osmotic shock with 10 mM CaCl 2 . Arrow indicates application of hypo-osmotic shock. White numbers show times (s) from application of hypo-osmotic shock. Solid lines show Ca 2+ change in the cytoplasm (red) and the nucleus (blue) and cell volume (black). Dashed lines show the start of increase in Ca 2+ level. Scale bars indicate 2 μm. ( b ) Time-lapse observation of WT and msy1 – msy2 – cells upon hypo-osmotic shock with BAPTA. Cells expressing EGFP were incubated in EMM2 medium supplemented with 1.2 M sorbitol and diluted 20-fold with 10 mM BAPTA. Photographs are displayed for every 10 s after the dilution (top). Relative cell volume changes in WT and msy1 – msy2 – cells are shown by solid and dashed lines, respectively (bottom). An arrow shows the application of hypo-osmotic shock. Scale bars indicate 2 μm. Full size image Msy1 regulates [Ca 2+ ] i increase on hypo-osmotic shock We then examined the influence of extracellular Ca 2+ in the hypo-osmotic shock response. When msy1 – msy2 – cells were subjected to hypo-osmotic shock with 10 mM CaCl 2 solution instead of distiled water, viability was decreased down to 8.6±11.6% in 30 min, which was significantly less than that in distiled water (51.4±9.0%) ( Fig. 6a ). Note that YES medium contains 120 μM Ca 2+ as measured by inductively coupled plasma-atomic emission spectrometry, and thus the Ca 2+ concentration after 20-fold dilution in distiled water is 6 μM. The effect of CaCl 2 was reversed when msy1 – msy2 – cells were transferred to a solution containing 10 mM BAPTA (86.6±6.3%). An improved survival rate was also observed when the cells were transferred to solutions containing NaCl, KCl, MgCl 2 or BaCl 2 . Interestingly, MnCl 2 , which can replace the functions of Ca 2+ (ref. 31 ), decreased viability upon hypo-osmotic shock, as with CaCl 2 . The viability of msy1 – msy2 – cells was decreased as the CaCl 2 concentration in the hypo-osmotic solution was increased, whereas that of WT, msy1 – and msy2 – cells was not changed ( Fig. 6b ). This observation indicates that the decrease in viability is dependent on extracellular Ca 2+ in msy1 – msy2 – cells. 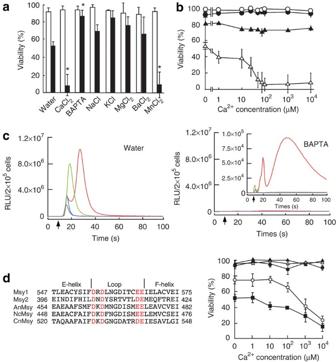Figure 6: The influence of Ca2+on the phenotype ofmsy1–msy2–cells. (a) The viability of WT (white bar) andmsy1–msy2–cells (black bar) after they were immersed in hypo-osmotic solution containing various substances and incubated for 30 min. *, Student'st-test,P<0.05 versus water. (b) The relationship between viability and Ca2+concentration in hypo-osmotic solution. Cells were immersed in hypo-osmotic solution containing various concentrations of CaCl2and incubated for 30 min: WT (closed circle),msy1–(open circle),msy2–(closed triangle) andmsy1–msy2–(open triangle). (c) Measurement of a Ca2+transient with aequorin. Cells of WT (blue),msy1–(green),msy2–(purple) andmsy1–msy2–(red) were subjected to hypo-osmotic shock with distiled water (left) and 10 mM BAPTA (right). Arrows represent the application of hypo-osmotic shock. An inset shows the graph in expanded vertical scale. (d) Conserved EF hand-like motif in fungal Msy1 homologues (left). An:Aspergillus nidulans, Nc:Neurospora crassa, Cn:Cryptococcus neoformans. The effect of a mutation in an EF hand-like motif of Msy1 and Msy2 (right). Themsy1–msy2–mutant was transformed with a plasmid bearing one of the genes encoding the following proteins: Msy1 (closed circle), Msy2 (closed triangle), mutant Msy1 (open circle), mutant Msy2 (open triangle) and empty vector (closed square). All of the data are means±s.d. from three independent experiments. Figure 6: The influence of Ca 2+ on the phenotype of msy1 – msy2 – cells. ( a ) The viability of WT (white bar) and msy1 – msy2 – cells (black bar) after they were immersed in hypo-osmotic solution containing various substances and incubated for 30 min. *, Student's t -test, P <0.05 versus water. ( b ) The relationship between viability and Ca 2+ concentration in hypo-osmotic solution. Cells were immersed in hypo-osmotic solution containing various concentrations of CaCl 2 and incubated for 30 min: WT (closed circle), msy1 – (open circle), msy2 – (closed triangle) and msy1 – msy2 – (open triangle). ( c ) Measurement of a Ca 2+ transient with aequorin. Cells of WT (blue), msy1 – (green), msy2 – (purple) and msy1 – msy2 – (red) were subjected to hypo-osmotic shock with distiled water (left) and 10 mM BAPTA (right). Arrows represent the application of hypo-osmotic shock. An inset shows the graph in expanded vertical scale. ( d ) Conserved EF hand-like motif in fungal Msy1 homologues (left). An: Aspergillus nidulans , Nc: Neurospora crassa , Cn: Cryptococcus neoformans . The effect of a mutation in an EF hand-like motif of Msy1 and Msy2 (right). The msy1 – msy2 – mutant was transformed with a plasmid bearing one of the genes encoding the following proteins: Msy1 (closed circle), Msy2 (closed triangle), mutant Msy1 (open circle), mutant Msy2 (open triangle) and empty vector (closed square). All of the data are means±s.d. from three independent experiments. Full size image The above result suggests that a lethal level of excessive Ca 2+ influx occurs in msy1 – msy2 – cells at a high CaCl 2 concentration. In fact, an excessive elevation in [Ca 2+ ] i under stress conditions is known to cause apoptosis-like cell death in yeast [32] . Thus, we measured quantitatively the change in [Ca 2+ ] i using aequorin to examine whether [Ca 2+ ] i was increased in msy1 – msy2 – cells upon hypo-osmotic shock. When WT, msy1 – and msy2 – cells were subjected to hypo-osmotic shock, a single Ca 2+ transient was generated as reported previously [12] , and msy1 – cells displayed a Ca 2+ transient greater than WT ( Fig. 6c ). By contrast, msy1 – msy2 – cells produced Ca 2+ transients with a shoulder and two peaks and the level of the second peak was approximately twofold higher than that of WT cells. The temporal pattern of the [Ca 2+ ] i changes suggests that the first peak in msy1 – msy2 – cells corresponds to the single peak in WT cells. We then examined the influence of the chelation of extracellular Ca 2+ using 10 mM BAPTA. In WT cells, 10 mM BAPTA dramatically decreased the Ca 2+ transient to leave only ~10 −4 -fold of that of the control ( Fig. 6c ). By contrast, the Ca 2+ transients of msy1 – msy2 – cells were decreased only ~10 −2 -fold following addition of BAPTA and were ~10-fold higher than the Ca 2+ transient of WT in the presence of BAPTA. We noted that BAPTA significantly retarded the generation of the weak peaks in both WT and mutant cells. The results with BAPTA suggest that approximately 90% or more of the Ca 2+ increase was supplied by the influx of extracellular Ca 2+ in WT and mutant cells. Given that fungal MscS homologues have a conserved EF hand-like motif ( Fig. 6d ), it is possible that [Ca 2+ ] i is detected by this motif. This possibility was examined by disrupting the motif of Msy1 and Msy2, and all glutamate and aspartate residues in the motif were replaced by alanine. When the mutant Msy1 was expressed under the nmt41 promoter in the msy1 – msy2 – mutant, viability still decreased in a Ca 2+ -dependent manner, whereas the expression of the intact Msy1 completely restored the viability to the WT levels ( Fig. 6d ). On the other hand, the mutant Msy2 suppressed the msy1 – msy2 – phenotype, like the intact Msy2. These findings suggest that the EF hand-like motif of Msy1 is involved in the detection of Ca 2+ concentration increases upon hypo-osmotic shock. Msy1 functions as a mechanosensitive channel To elucidate whether Msy1 and Msy2 function as mechanosensitive channels, we expressed the msy1 + and msy2 + genes in E. coli spheroplasts lacking both mscS and mscK and examined mechanosensitive channel activity using the inside-out, excised patch-clamp technique. When an increasing negative pressure was applied to the patch membrane through the patch pipette, a current with approximately 0.25 nS in conductance was observed in Msy1-expressing spheroplasts ( n =9/28) ( Fig. 7a ). A further increase in the negative pressure opened E. coli MscL, which has a conductance of approximately 3 nS. Only the channel activity of MscL was detected in spheroplasts harbouring an empty vector ( n =10/10). The conductance of Msy1 was 0.25±0.05 nS ( Fig. 7b ). Voltage-dependent rectification, which is a property of MscS, was not observed in Msy1. This may be due to loss of positive charge at the position that corresponds to MscS K169 ( Fig. 1c ), which contributes noticeably to the rectification of MscS [33] . On the other hand, the channel activity of Msy2 was not detected under the same experimental conditions for an unknown reason. We found that MscS, but not Msy1 and Msy2, rescued E. coli MJF612 cells [34] lacking MscM, MscK, MscS and MscL from hypo-osmotic shock-induced cell lysis ( Fig. 7c ). 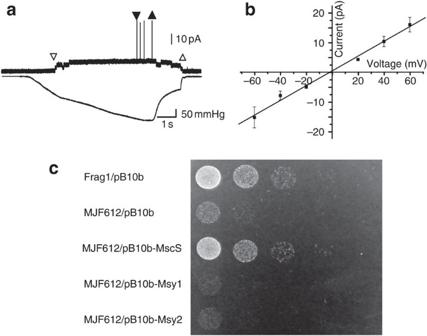Figure 7: Electrophysiological characterization of Msy1. (a) Single channel recording at +20 mV of pipette potential in Msy1-expressingE. colispheroplasts. Upper trace shows the current. Lower trace shows the amplitude of pressure applied to the patch membrane. The opening and closing of channels are shown by downward and upward triangles, respectively: Msy1 (open triangle),E. coliMscL (closed triangle). (b) Current–voltage relationship of Msy1. Channel conductance calculated from the regression line is 0.25±0.05 nS. All of the data are means±s.d. from three independent experiments. (c) Osmotic-shock assay ofE. colicells expressing Msy1 and Msy2. Strains, Frag1 (F′,rha,thi,gal,lacZ) and MJF612 (Frag1 ΔmscL::cm, ΔmscS, ΔmscK::kan, ΔybdG::apr), were cultured in LB medium, and adapted in LB medium containing 475 mM NaCl. Hypo-osmotic shock was performed by 20-fold dilution into LB medium. Serial dilutions were plated on LB with ampicillin plate and incubated overnight. Figure 7: Electrophysiological characterization of Msy1. ( a ) Single channel recording at +20 mV of pipette potential in Msy1-expressing E. coli spheroplasts. Upper trace shows the current. Lower trace shows the amplitude of pressure applied to the patch membrane. The opening and closing of channels are shown by downward and upward triangles, respectively: Msy1 (open triangle), E. coli MscL (closed triangle). ( b ) Current–voltage relationship of Msy1. Channel conductance calculated from the regression line is 0.25±0.05 nS. All of the data are means±s.d. from three independent experiments. ( c ) Osmotic-shock assay of E. coli cells expressing Msy1 and Msy2. Strains, Frag1 (F′, rha , thi , gal , lacZ ) and MJF612 (Frag1 Δ mscL :: cm , Δ mscS , Δ mscK :: kan , Δ ybdG :: apr ), were cultured in LB medium, and adapted in LB medium containing 475 mM NaCl. Hypo-osmotic shock was performed by 20-fold dilution into LB medium. Serial dilutions were plated on LB with ampicillin plate and incubated overnight. Full size image We have demonstrated that two fission yeast MscS homologues, Msy1 and Msy2, have an essential role in the hypo-osmotic shock response through modulating [Ca 2+ ] i and cell volume. The cell volume of the msy1 – msy2 – double mutant was increased to a level greater than that of WT cells (that is, overshoot), and then decreased. The cell volume increase was accompanied by elevation of [Ca 2+ ] i mainly through the influx of extracellular Ca 2+ , and the elevated level was higher in msy1 – msy2 – cells than in WT cells. Importantly, msy1 – msy2 – cells, but not WT cells, eventually lost viability under these conditions. We postulate that critical roles of Msy1 and Msy2 are the modulation of [Ca 2+ ] i and cell volume leading to maintenance of viability, on the basis of the observations below. First, following hypo-osmotic shock with excess extracellular Ca 2+ , the viability of msy1 – msy2 – cells, but not of WT cells, was lowered. Second, when the hypo-osmotic shock-induced [Ca 2+ ] i elevation was restricted by approximately 90% by transferring msy1 – msy2 – cells to 10 mM BAPTA solution, the cells did not show a marked loss of viability. Therefore, it is likely that Msy1 and Msy2 function to prevent cell death by modulating [Ca 2+ ] i upon a sudden increase in cell volume. Cell volume regulation has been well studied in mammalian cells. Following hypo-osmotic shock, the cells swell quickly, but soon start recovering their volume near the original level by a mechanism called regulatory volume decrease (RVD) [28] . During this process, cell swelling induces a [Ca 2+ ] i increase that has a regulatory role for ion homoeostasis across the plasma membrane. Fission yeast seems to have a similar but distinct mechanism. WT cells of fission yeast swell in spite of having the cell wall, but maintain a plateaued swollen level. By contrast, msy2 – and msy1 – msy2 – cells showed a transient overshoot of the cell volume increase. Msy2 may be a major mediator of cell volume regulation that does not utilize an RVD-like mechanism. Another difference in cell volume regulation between mammalian and fission yeast cells is the localization of ion channels and transporters involved in this process. It is widely accepted that mammalian cell volume regulation is governed by ion channels and transporters in the plasma membrane that are responsible for the fluxes of K + and Cl − as well as Ca 2+ (see Okada et al . [28] ). This is also true for bacterial cells [5] . By contrast, our study has shown that Msy1 and Msy2 are localized in organellar membranes: Msy1 is localized mainly in the perinuclear ER and Msy2 in the cortical ER. This localization examined by tagged Msy1 and Msy2, however, cannot exclude the possibility that intact Msy1 and Msy2 are present in the plasma membrane. As the [Ca 2+ ] i elevation following hypo-osmotic shock was greater in msy1 – and msy1 – msy2 – cells than in WT cells, the primary function of Msy1 could be to stimulate the efflux and/or sequestration of the excess Ca 2+ from the cytoplasm. If this function is impaired, excess Ca 2+ should result in cell death. As Msy1 is a mechanosensitive channel, it is possible that it senses membrane stretch and activates organellar and plasma-membrane Ca 2+ -ATPases and/or vacuolar H + /Ca 2+ exchangers to lower abnormally high [Ca 2+ ] i by an-as-yet unidentified mechanism. On the other hand, Msy2 probably contributes to [Ca 2+ ] i elevation for volume regulation because the msy2 − mutant displays a lower [Ca 2+ ] i elevation and a greater volume increase upon hypo-osmotic shock than WT. Thus, we suppose that Ca 2+ efflux from the cortical ER through Msy2 activates a Ca 2+ -activated cell volume regulator. Msy1 and Msy2 have differential functions in [Ca 2+ ] i elevation and volume regulation, though their mechanistic roles should be tested in future studies. Although the low-viability phenotype of msy1 – msy2 – cells is suppressed by individual overexpression of msy1 + and msy2 + , we suspect that Msy1 and Msy2 act in sequence in the hypo-osmotic shock response. Upon hypo-osmotic shock, msy2 – cells lose viability significantly ( Fig. 4b ), and exhibit a greater and longer volume increase than msy1 – cells ( Fig. 4a ), suggesting that Msy2 functions in cell volume regulation. On the other hand, msy1 − cells show a larger and longer [Ca 2+ ] i increase than WT and msy2 – cells, suggesting that Msy1 is involved in the removal of cytoplasmic Ca 2+ . If the function of Msy1 is to restrict the elevation of [Ca 2+ ] i to a moderate level, it is possible that this protein can monitor the intracellular Ca 2+ concentration. Consistent with this idea, an Msy1 derivative with a disrupted EF hand-like motif failed to suppress the phenotype of msy1 – msy2 – cells. Disruption of the EF hand-like motif of Msy2 did not have a similar effect. This motif is conserved in fungal MscS homologues, in contrast to its absence in MscS homologues of plants and algae. Because the levels of msy1 + and msy2 + transcripts were upregulated by both hyper- and hypo-osmotic shocks, fungal MscS homologues would sense not only membrane stretch but also intracellular Ca 2+ levels in response to both shocks. A unique feature of Msy1 and Msy2 as members of the MscS family is that they are localized in the perinuclear and cortical ERs, respectively. In Arabidopsis , in contrast, MSL2 and MSL3 are localized in the chloroplast membrane and several other MscS-like proteins in the plasma membrane [10] , [35] . The function of the chloroplast MscS-like proteins is to regulate chloroplast shape [10] and to protect plastids from hypo-osmotic stress during normal plant growth [36] . In Chlamydomonas , MSC1 is present as punctuate spots in the chloroplast and cytoplasm and involved in chlorophyll localization [11] . Thus, our study adds a new aspect of the MscS family in terms of its localization and function. In summary, we propose that Msy1 and Msy2 regulate [Ca 2+ ] i and cell volume in the hypo-osmotic shock response. Hypo-osmotic shock causes cell swelling, which activates Msy1 and Msy2 in the perinuclear and cortical ERs. Cell swelling also promotes the [Ca 2+ ] i increase that can be suppressed by activated Msy1. Regulation of the [Ca 2+ ] i increase and cell volume by Msy1 and Msy2 is essential for maintenance of viability upon hypo-osmotic shock. Microbial strains and culture conditions S. pombe strain FY15952 ( h – ade6-M210 leu1-32 ura4-D18 ) was used as the wild type. YN001 ( msy1 :: ura4 + in FY15952), YN002 ( msy2 :: kanMX6 in FY15952), YN003 ( msy1 :: ura4 + msy2 :: kanMX6 in FY15952) and YN004 ( msy1 + - 4HA in FY15952) were created in this study. Cells were cultured at 30 °C in rich medium (YES) or synthetic medium (EMM2) [37] . E. coli strain PB113 (Δ mscs Δ msck ) was used for the electrophysiological experiment [38] . Strains Frag1 (F′ rha thi gal lacZ ) and MJF612 (Δ mscL :: cm Δ mscS Δ mscK :: kan Δ ybdG :: apr in Frag1) were used for osmotic-shock assays [34] . XL1-Blue (Stratagene) was used for cloning. Gene cloning A Blast search for E. coli MscS was performed using the S. pombe GeneDB ( http://www.genedb.org/genedb/pombe/ ). Systematic Names: SPCC1183.11 and SPAC2C4.17c were found as homologues of MscS at a threshold E -value of 0.01 and designated Msy1 and Msy2, respectively. msy1+ and msy2+ were amplified by PCR with KOD -plus- DNA polymerase (Toyobo) from a complementary DNA (cDNA) library, pTN-RC5, which was provided by RIKEN BRC through the National Bio-Resource Project of MEXT, Japan. The open reading frames (ORFs) of msy1 + and msy2 + were cloned into the pGEM-T easy vector (Promega) and sequenced with ABI3130 (Applied Bio Instrument). TMHMM ( http://www.cbs.dtu.dk/services/TMHMM/ ) and PROSITE ( http://au.expasy.org/prosite/ ) were used to predict secondary structure. Gene disruption and integration Yeast gene disruption and integration were performed by the lithium acetate method [39] . FY15952 was used as a parental strain for all mutants. Strains carrying msy1 :: ura4 + and msy2 :: kanMX6 genomic replacements were created by the insertion of a ura4 -marker cassette in the Bam HI /Nru I site and a kanMX6 -marker cassette in the Blp I/ Nhe I site, respectively. Msy1-4HA was constructed by gene integration with four HA tags at the carboxyl terminus. Plasmid construction The yeast expression vectors pREP1, pREP2, pREP41 and pREP42 were used [40] . The ORFs of msy1 + and msy2 + were inserted into the Sal I/ Not I site of pREP41. The ORFs of msy1 + tagged with three HA antigens at the C-terminus and msy2 + tagged with mCherry at the N-terminus were inserted into the Sal I/ BamH I site of pREP41. These plasmids were used for complementation experiments. The ORFs of pma1 + and rtn1 + tagged with EGFP at the C-terminus and msy2 + tagged with mCherry at the N-terminus were inserted into the Sal I/ BamH I site of pREP41 and pREP42. These plasmids and pREP41-Calnexin-EGFP were used for fluorescent microscopic observations. The ORFs of EGFP and yellow Cameleon-nano15 were cloned into the Sal I/ Xma I site of pREP1. The ORF of apoaequorin was inserted into the Sal I/ Sma I site of pREP1. To substitute all glutamate and aspartate in the EF hand-like motif of Msy1 and Msy2 to alanine, point mutations were introduced into the EF hand-like motif of Msy1 and Msy2 in pREP41 using the site-directed mutagenesis kit (Toyobo) according to the manufacturer's instructions. Quantitative RT–PCR The cells were exposed to osmotic shock with YES medium containing 1.2 M sorbitol and distiled water for 30 min. Approximately 3×10 7 cells were prepared and total RNA was extracted with a FastPure RNA kit (Takara, Shiga). Aliquots of 400 ng of RNA were reverse-transcribed with Primescript reverse transcriptase (Takara, Shiga using random hexamers and an oligo-d(T) primer. Real-time PCR was performed through 40 cycles of 95 °C for 5 s and 60 °C for 30 s using the thermal cycler Dice (Takara, Shiga). The gene-specific primers were designed to amplify a cDNA fragment of between 120 and 200 bp and listed in Supplementary Table S1 . The specificity of the PCR using SYBR premix ExTaq (Takara, Shiga) was evaluated by melting curve analysis and electrophoresis. The amount of RNA was calculated according to the manufacturer's protocol and normalized to that of histidinol-phosphate aminotransferase 3 (His3) mRNA, as its expression is unaffected by osmotic shock. Measurement of viability upon hypo-osmotic shock Cells were grown to 1×10 7 cells per ml in YES medium. The medium was supplemented with an equal volume of YES or EMM2 medium with 2.4 M sorbitol and incubated at 30 °C for 4 h. The culture was diluted 20-fold with distiled water, as hypo-osmotic shock. After 30-min incubation at 30 °C, viability was examined with methylene blue as described previously [41] , and the ratio of the number of cells alive ( N alive ) to that counted ( N all ) was used to calculate viability ( N alive / N all ). Time-lapse imaging of S. pombe cells Yeast cells harbouring pREP1-EGFP (S65T) and yellow Cameleon-nano15 were grown to 1×10 7 cells per ml in EMM2 medium for the measurement of cell volume and cytosolic Ca 2+ imaging, respectively. To the cell culture was added an equal volume of EMM2 medium supplemented with 2.4 M sorbitol (final: 1.2 M) and incubated for 4 h. Yeast cells were placed on a poly-l-lysine-coated glass-bottomed dish (Matsunami, Osaka), and diluted 20-fold with distiled water or 10 mM CaCl 2 , as hypo-osmotic shock. Microscopy was performed with a microscope (Axiovert 200M; Carl Zeiss Japan, Tokyo) and a Plan-Neofluar X100/NA 1.30 oil immersion objective (Carl Zeiss Japan, Tokyo). Pictures were acquired at room temperature with a CCD camera (CoolSNAP; Nippon Roper, Tokyo) using MetaMorph and Metavue software (Molecular Device, Tokyo). The DualView beam splitter (Molecular Device, Tokyo) was used for F 528 / F 488 ratio imaging. The fluorescent area of two-dimensional images was measured to evaluate cell volume. Immunolabeling Whole-cell extracts were prepared from fission yeast cells in the exponential phase. The cells were suspended in lysis buffer (50 mM Tris–HCl, pH 8.0, 0.1% Triton X-100, 0.5% SDS and 2 mM PMSF) and vortexed at 4 °C for 15 min in the presence of glass beads (Sigma). After centrifugation, the supernatant was mixed with an equal volume of 2× SDS sample buffer and boiled at 95 °C for 5 min. Proteins were separated on an 8% SDS–polyacrylamide gel electrophoresis (SDS–PAGE) gel and electrotransferred to a PVDF membrane (Bio-Rad). The membrane was blocked with Blocking-One (Toyobo) for 1 h, incubated with the anti-HA mouse monoclonal antibody (12CA5) (1:3,000), anti-c-myc rabbit antibody (Sigma) (1:3,000), anti-FLAG mouse antibody (Sigma) (1:6,000), anti-Pma1 rabbit antibody (1:500), suspended in Can Get Signal 1 solution (Toyobo) for 1 h at room temperature, and then incubated with secondary antibody (HRP-conjugated anti-mouse IgG and HRP-conjugated anti-rabbit IgG, GE Healthcare) in Can Get Signal 2 solution (1:20,000) for 1 h. The secondary antibody was detected with an Immobilon Western Chemiluminescent HRP Substrate kit (Millipore) according to the manufacturer's directions. Fluorescence microscopy Localization within cells expressing pSM-Bip-myc-ADEL was detected by indirect immunofluorescence, according to the method described previously with slight modifications [42] . Briefly, cells were fixed with 3% formaldehyde (EM grade, TAAB) at 30 °C for 90 min in YES medium, and washed twice with PEM (100 mM PIPES, 1 mM EGTA, 1 mM MgSO 4 , pH 6.9). Cell walls were digested with 0.5 mg ml −1 Zymolyase-100T (SEIKAGAKU CORPORATION, Japan) in PEMS (100 mM PIPES, 1 mM EGTA, 1 mM MgSO 4 , 1.2 M sorbitol, pH 6.9) at 37 °C for 1 h. The cells were permeabilized with 1% Triton X-100 for 15 min and washed three times with PEM. The cells were blocked with PEMBAL (100 mM PIPES, 1 mM EGTA, 1 mM MgSO 4 , 100 mM lysine hydrochloride, 1% BSA, 0.1% NaN 3 , pH 6.9) for 1 h. Anti-HA mouse monoclonal antibody (12CA5) (Funakoshi) and anti-c-myc rabbit antibody (Sigma) were used for the primary antibody solution at 1:300 dilutions with PEMBAL. Alexa488-conjugated anti-mouse IgG (Life Technologies Japan, Tokyo) and Alexa546-conjugated anti-rabbit IgG (Life Technologies Japan, Tokyo) were used as the secondary antibody at 1:400 dilutions. The nucleus was detected with 50 ng ml −1 DAPI. All procedures were carried out at room temperature and, where appropriate, with protection from light. Immunolabeled cells were observed under an ELYRA superresolution microscope (Carl Zeiss Japan, Tokyo). Hoechst33342, EGFP and mCherry were observed with a TSC-SPE confocal microscope (Leica Microsystems Japan, Tokyo). Subcellular fractionation Yeast cell extracts, prepared from 2×10 8 cells harbouring pREP2-Msy2-3FLAG and pSM-BiP-myc-ADEL, were subjected to subcellular fractionation by sucrose density gradient centrifugation, according to the method described by Egner et al . [43] . After centrifugation, proteins in each fraction were precipitated with 10% trichloroacetic acid, washed twice with cold acetone and dissolved in SDS–sample buffer. The separated samples were subjected to SDS–PAGE and immunoblotting. Measurement of [Ca 2+ ] i with aequorin Cells harbouring pREP1-apoaequorin were grown to the early logarithmic phase in EMM2 medium. Cells were harvested by centrifugation and resuspended in fresh EMM2 medium supplemented with 1.2 M sorbitol and 15 μM coelenterazine. To convert apoaequorin to aequorin, the cells were incubated for 4 h at 30 °C and then washed three times with fresh EMM2 supplemented with 1.2 M sorbitol. The cells were resuspended to 10 7 cells per ml in EMM2 supplemented with 1.2 M sorbitol. The light emission levels as relative light units were measured using the lumicounter2500 (MICROTEC, Chiba) at 1 s intervals. Electrophysiology Giant spheroplasts were obtained from E. coli cells harbouring the expression vector pB10b as described previously [44] . Gene expression was induced at 37 °C for 3 h. Single-channel currents were recorded from inside-out excise patches from the giant spheroplasts. The pipette solution contained 200 mM KCl, 40 mM MgCl 2 , 10 mM CaCl 2 , 0.1 mM EDTA and 5 mM HEPES-KOH (pH 7.2). The bath solution consisted of the pipette solution supplemented with 300 mM sucrose to stabilize the spheroplasts. Currents were amplified using an Axopatch 200B amplifier (Molecular Devices, California) and filtered at 2 kHz. Current recordings were digitized at 5 kHz using a Digidata 1322A interface with pCLAMP9 software (Molecular Devices, California). Negative pressure was applied by syringe-generated suction through the patch-clamp pipette and measured with a pressure gauge. Osmotic-shock assays E. coli strains, Frag1 and MJF612, were cultured overnight in LB medium with ampicillin, and transferred to LB medium supplemented with 500 mM NaCl by 20-fold dilution (final concentration, 475 mM NaCl). After incubation at 37 °C for 2 h, gene expressions were induced for 30 min by 1 mM IPTG at 37 °C, and then diluted 1:20 into LB medium prewarmed at 37 °C. Cells were serially diluted 10-fold and aliquots were plated on LB with ampicillin plates. How to cite this article: Nakayama, Y. et al . Organellar mechanosensitive channels in fission yeast regulate the hypo-osmotic shock response. Nat. Commun. 3:1020 doi: 10.1038/ncomms2014 (2012).